Plant genomes enclose footprints of past infections by giant virus relatives Nucleocytoplasmic large DNA viruses (NCLDVs) are eukaryotic viruses with large genomes (100 kb–2.5 Mb), which include giant Mimivirus, Megavirus and Pandoravirus. NCLDVs are known to infect animals, protists and phytoplankton but were never described as pathogens of land plants. Here, we show that the bryophyte Physcomitrella patens and the lycophyte Selaginella moellendorffii have open reading frames (ORFs) with high phylogenetic affinities to NCLDV homologues. The P. patens genes are clustered in DNA stretches (up to 13 kb) containing up to 16 NCLDV-like ORFs. Molecular evolution analysis suggests that the NCLDV-like regions were acquired by horizontal gene transfer from distinct but closely related viruses that possibly define a new family of NCLDVs. Transcriptomics and DNA methylation data indicate that the NCLDV-like regions are transcriptionally inactive and are highly cytosine methylated through a mechanism not relying on small RNAs. Altogether, our data show that members of NCLDV have infected land plants. Viruses are environmentally ubiquitous, obligate intracellular parasites that infect organisms from all three superkingdoms. In addition to their role in major evolutionary transitions [1] , [2] and control over host populations, viruses can become an inherent part of the genetic material of their host through horizontal gene transfer (HGT). These integrated viral sequences, referred to as endogenous viral elements [3] , are of particular interest as they constitute footprints of past infections that can reveal the nature of as yet unidentified extant or ancient viruses and help to reconstruct scenarios of host–virus co-evolution [4] , [5] . The nucleocytoplasmic large DNA viruses (NCLDVs) form one of the largest divisions of the virus kingdom [6] , [7] . They are characterized by either a cytoplasmic or nucleo-cytoplasmic replication cycle [6] , [8] and the largest known genomes in the viral world (100 kb–2.5 Mb double-strand DNA (dsDNA)), a conspicuous characteristic that led scientists to dub them ‘giant viruses’ or ‘giruses’ [9] . This group of apparently monophyletic viruses comprises at least six formally recognized families: Poxviridae , Asfarviridae , Iridoviridae , Ascoviridae , Phycodnaviridae and Mimiviridae [10] . In addition, Marseillevirus [11] , the related Lausannevirus [12] , and the more recently discovered Pandoravirus [13] could not be assigned to any of the above families, and are likely to become founding members of two new families. The complexity of NCLDVs in terms of genome size, particle size and metabolic capabilities (such as their role in photosynthesis and apoptosis) has challenged many concepts in virology [14] . Furthermore, viruses in the Mimiviridae family encode genes involved in translational activity, a metabolism that was considered as an exclusivity of cellular organisms. Collectively, NCLDVs are known to infect animals and diverse unicellular eukaryotes [15] but were never described as pathogens of land plants (that is, Embryophyta ). The specific avoidance of land plants as hosts remains unclear. It may be the consequence of unique defense mechanisms that allow land plants to escape this type of pathogen or inability for NCLDVs to develop a successful infection cycle in land plants. Alternatively, unknown members of NCLDV may be pathogens of land plants, but their existence has never been discovered until now. Endogenized Phycodnaviridae genome segments, of recent origin, have been identified in the nuclear genomes of diverse algal groups including the brown algae Ectocarpus siliculosus [16] and Feldmannia species [17] , the haptophyte Emiliania huxleyi [18] and the green alga Chlorella variabilis [19] . Here we analysed 13 sequenced land plant genomes to search for the presence of DNA regions that possibly originated from NCLDVs. We report the identification of several loci in the genomes of the early diverging plants S. moellendorffii and P. patens , which suggests that their progenitors were infected by NCLDVs at some point in the evolution of their lineages. Phylogenetic and genome reconstructions support the hypothesis that the P. patens donor viruses define a new family among the NCLDVs. NCLDV homologues in plant genomes The full complement of predicted proteins from 13 fully sequenced plant species were used to probe the NCBI database using BLASTP ( E -value <1e−5). For each protein query, the alignment scores with the best non-NCLDV hit (with exclusion of species in the same taxonomical family as the query sequence) and the best NCLDV hit were recorded. BLAST scores were then normalized by the score of the alignment of the query sequence against itself (that is, self-score), resulting in relative scores expressed in percent of self-score. The number of plant proteins with both NCLDV and non-NCLDV hits ranged from 2,662 for P. patens to 5,431 for P. abies . Non-NCLDV hit scores were plotted against NCLDV hit scores in Fig. 1 and Supplementary Fig. 1 . 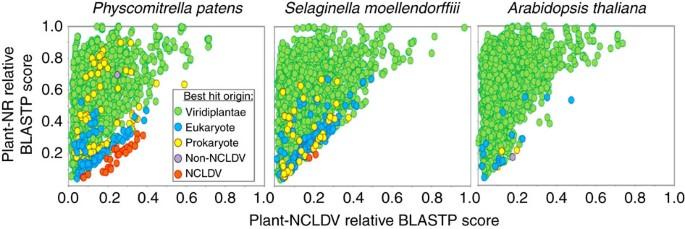Figure 1: Similarity plot of plant proteins against their closest homologues in viruses and non-redundant (NR) database. Circles represent relative BLASTP scores of plant proteins aligned against their best hits in the NR database (yaxis; with exclusion of hits originating from NCLDV and organisms in the same taxonomic family as the query) and the NCLDV section of NR (xaxis). BLAST scores were normalized by dividing them by the score of the alignment of the query sequence against itself. Circles were coloured according to the origin of the best scoring hit (Non-NCLDV refers to viruses out of the NCLDV division). The results for 3 representative plants out of the 13 studied species are shown here. The similarity plot forArabidopsis thalianais characteristic of the ten other studied embryophytes. Figure 1: Similarity plot of plant proteins against their closest homologues in viruses and non-redundant (NR) database. Circles represent relative BLASTP scores of plant proteins aligned against their best hits in the NR database ( y axis; with exclusion of hits originating from NCLDV and organisms in the same taxonomic family as the query) and the NCLDV section of NR ( x axis). BLAST scores were normalized by dividing them by the score of the alignment of the query sequence against itself. Circles were coloured according to the origin of the best scoring hit (Non-NCLDV refers to viruses out of the NCLDV division). The results for 3 representative plants out of the 13 studied species are shown here. The similarity plot for Arabidopsis thaliana is characteristic of the ten other studied embryophytes. Full size image As expected the large majority of plant proteins had their best matches in plant and eukaryotic homologues (that is, green and blue dots in Fig. 1 and Supplementary Fig 1 ) than with NCLDV homologues. Furthermore, all plants but V. vinifera also had some best matches in prokaryotes or non-NCLDV viruses (mostly retro-transcribing viruses, that is, yellow and purple dots) that likely reflect DNA contamination or HGTs. Interestingly, the bryophyte P. patens and lycophyte S. moellendorffii genomes encoded a number of proteins that had best matches with NCLDV homologues (red dots), suggesting that they were more closely related to their NCLDV counterparts than to plant sequences. However, the best alignment score criterion alone cannot be taken as a demonstration of HGT or close evolutionary relationship. Nevertheless, sequence similarity measures can be used for scanning large amounts of data and identify potential protein candidates for further analysis. Hereafter, plant sequences that had a best match in NCLDV are referred to as NCLDV-like genes or proteins. S. moellendorffii NCLDV-like genes Two predicted S. moellendorffii proteins, including one of unknown function (Genbank accession no. EFJ10148 ) and a putative exoribonuclease (EFJ26844), had a best relative score with an NCLDV protein. For each of these two proteins, additional unannotated proteins were identified by scanning the S. moellendorffii genome using TBLASTN searches with the NCLDV-like proteins as the query. When significant hits were identified, the GENEWISE (ref. 20 ) software was used to predict the open reading frames (ORFs). We examined the evolutionary relationship of the two lycophyte protein families with their NCLDV homologues using maximum likelihood (ML) phylogenetic reconstruction. Protein EFJ10148 had homologues with significant similarity (BLASTP E -value <1e−5) in a small number of fungi and in a single NCLDV member, namely Acanthocystis turfacea Chlorella virus NE-JV-2, a phycoDNAvirus that infects a green alga. As shown in Fig. 2a and Supplementary Fig. 2 , the corresponding ML tree did not confirm monophyly between NE-JV-2 and Selaginella proteins. Thus, although they were likely acquired horizontally, no conclusion could be drawn regarding the exact origin of the corresponding Selaginella genes. In contrast, S. moellendorffii putative exoribonucleases had homologues in many cellular organisms including plants, as well as in several members of NCLDVs. ML phylogenetic reconstruction confirmed closest evolutionary relationships between lycophyte proteins and NCLDVs comprising organic lake phycoDNAviruses, Phaeocystis globosa virus and Cafeteria roenbergensis virus ( Fig. 2b and Supplementary Fig. 3 ). This result is consistent with the hypothesis that the S. moellendorffii exoribonuclease genes have a viral origin and were acquired through HGT. This also suggests that a Selaginella ancestor had physical contacts with an unknown member of NCLDVs. Further analysis in the immediate vicinity of the two gene families failed to identify additional NCLDV-like genes. 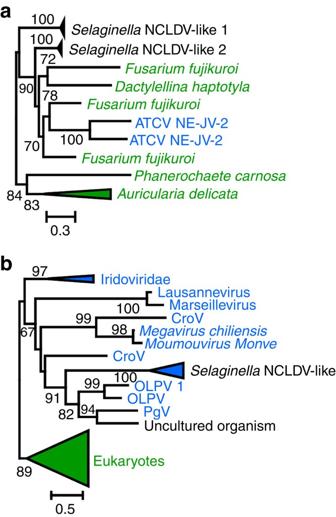Figure 2: Phylogenetic trees ofS. moellendorffiiNCLDV-like proteins. (a) Maximum likelihood (ML) tree of the unknown protein (EFJ10148). (b) ML tree of the exoribonuclease (EFJ26844). NCLDV and eukaryotic sequence names are shown in blue and green, respectively. For clarity, subtrees containing sequences originating from the same taxonomic clade were condensed (coloured triangles). Statistical supports for branch in percent (approximate likelihood ratio test) are shown beside nodes (only branch supports >50%). Scale bar represents the number of substitutions per amino-acid site. ATCV,Acanthocystis turfacea chlorellavirus; CroV,Cafeteria roenbergensisvirus; OLPDV, organic lake Phycodnavirus; PgV,Phaeocystis globosavirus. Figure 2: Phylogenetic trees of S. moellendorffii NCLDV-like proteins. ( a ) Maximum likelihood (ML) tree of the unknown protein (EFJ10148). ( b ) ML tree of the exoribonuclease (EFJ26844). NCLDV and eukaryotic sequence names are shown in blue and green, respectively. For clarity, subtrees containing sequences originating from the same taxonomic clade were condensed (coloured triangles). Statistical supports for branch in percent (approximate likelihood ratio test) are shown beside nodes (only branch supports >50%). Scale bar represents the number of substitutions per amino-acid site. ATCV, Acanthocystis turfacea chlorella virus; CroV, Cafeteria roenbergensis virus; OLPDV, organic lake Phycodnavirus; PgV, Phaeocystis globosa virus. Full size image P. patens NCLDV-like genes are physically clustered Investigation on the physical location of the P. patens NCLDV-like genes along with scaffolds revealed that they are clustered at a few discrete loci. These regions contained only a few predicted genes, presumably due to the difficulty for gene prediction programmes to predict non-plant genes in a plant DNA context. We manually reannotated the corresponding sequences using a standard ORFing strategy, which is convenient for virus genome annotation because virus genes are generally devoid of introns. Overall, 61 loci containing two or more ORFs were identified with sizes ranging from 2 to 34 kb ( Supplementary Fig. 4 ). Thirty additional smaller DNA stretches (<2 kb) containing truncated NCLDV-like ORFs were also identified but not characterized further. The cumulated size of the NCLDV-like regions slightly exceeded 561 kb (that is, 0.12% of the moss genome). The 61 loci exhibited high nucleotide similarity (>92% identity) between each other; including in intergenic regions. The gene order was generally conserved between regions except a few noticeable rearrangements including internal inversions and duplications as well as retrotransposon insertions ( Supplementary Fig. 4 ). These observations point to a common origin of the moss NCLDV-like regions. Based on the most common 2-by-2 gene arrangements found in the genome and average sizes of ORFs and intergenic regions (after exclusion of sequences containing retrotransposon sequences), a consensus structure for the NCLDV-like DNA was inferred ( Fig. 3 ). This consensus probably resembles the organization of the common ancestor of NCLDV-like regions. Overall, the reconstructed region spans over 13 kb and contains 20 original ORFs. None of the extant NCLDV-like regions contains a full complement of 20 ORFs. Instead, regions encoded different assortments of NCLDV-like genes containing 2–16 distinct gene families. 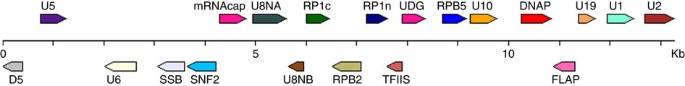Figure 3: Consensus structure of theP. patensNCLDV-like regions. Arrows represent individual ORFs and their transcriptional orientations. The consensus gene order was established based on the most common 2-by-2 gene arrangements found in the genome. Consensus sizes of ORFs and intergenic regions were determined based on average sizes of ORFs and intergenic regions in the genome assembly (after exclusion of sequences containing retrotransposon sequences). Figure 3: Consensus structure of the P. patens NCLDV-like regions. Arrows represent individual ORFs and their transcriptional orientations. The consensus gene order was established based on the most common 2-by-2 gene arrangements found in the genome. Consensus sizes of ORFs and intergenic regions were determined based on average sizes of ORFs and intergenic regions in the genome assembly (after exclusion of sequences containing retrotransposon sequences). Full size image The 20 gene families encoded 5 of the 31 proteins most consistently found in large dsDNA viruses (that is, ‘core’ genes [6] ; Table 1 and Supplementary Table 1 ). We identified 3 of the 9 most conserved (type I) core genes (including DNA polymerase (DNAP), D5 helicase-primase and D6/D11-like SNF2 helicase) and 2 out of the 14 type III (lesser conserved) core genes (that is, RP1 and RPB2, subunits of the DNA-dependent RNA polymerase (RNAP)). In addition, nine ORFs corresponding to gene families not initially classified in the NCLDV most conserved gene groups were conserved in various NCLDV families, including Flap endonuclease, Uracil-DNA glycosylase, mRNA capping methyltransferase, RNAP subunit 5 and 2, transcription elongation factor S-II, single-stranded DNA-binding (SSB) protein and two unknown proteins. Interestingly, two ORFs (RP1n and RP1c), respectively, encode the N and C terminals of a RNAP largest subunit (RP1). No NCLDV-like regions contained an intact copy of the original RP1 gene (that is, RP1n and RP1c encoded in a single ORF), suggesting that a fission of the RP1 gene occurred in the ancestor of moss NCLDV-like regions. This ‘split’ subunit structure is analogous to the organization of the archaeal large RNAP subunit that has also undergone gene fission [21] . Table 1 Plant NCLDV-like gene families. Full size table We took advantage of long-terminal repeat (LTR) retrotransposon (LTR-RT) insertions found within some NCLDV-like regions to estimate the minimal age of their insertions (see Methods). We calculated that LTR-RT insertions occurred within a range of 0.3–3.9 million years ago, suggesting that the corresponding NCLDV-like loci were acquired at least this long ago ( Supplementary Table 2 ). In agreement with this age estimation, PCR amplification demonstrated that NCLDV-like genes were also present in the genomes of two other P. patens ecotypes isolated in Germany and Switzerland ( Supplementary Fig. 5 ). P. patens NCLDV-like regions have a viral origin DNAP is the most commonly used phylogenetic marker for classification of large DNA viruses [22] , [23] . The ML phylogenetic tree of DNAP ( Fig. 4 and Supplementary Fig. 6 ) placed the NCLDV-like region products outside cellular clades, which include archaeal DNAP and eukaryotic DNAP alpha, delta and zeta. The genome of P. patens contains one or two paralogous copies for cellular DNAPs alpha, delta and zeta genes. However, the additional NCLDV-like DNAPs constituted a sister group to Lausannevirus and members of the Iridoviridae and Ascoviridae families. This topology is consistent with the hypothesis that the corresponding genes have a viral origin. As reported elsewhere [10] , ML phylogenetic reconstruction of DNAPs was unable to recover a monophyly for the NCLDV proteins. Instead NCLDV DNAP proteins formed a polyphyletic clade with eukaryotic DNAP delta and zeta. However, the apparent non-monophyly of the NCLDV DNAPs is likely erroneous and results from branch length effects, in particular, acceleration of evolution in some of the viruses resulting in long branch attraction [10] . Phylogenetic trees of the 11 other protein families consistently placed the moss NCLDV-like sequences among NCLDVs ( Fig. 4 and Supplementary Figs. 7–17 ). However, NCLDV-like proteins always emerged as a sister group to existing NCLDV families, suggesting that the NCLDV-like regions were possibly acquired from a NCLDV family distinct from the currently known NCLDV families. In six phylogenetic trees (that is, DNAP, D5, FLAP, SNF2, UDG and U10), the NCLDV-like proteins emerged next to Marseillevirus (and/or Lausannevirus), Iridoviridae and Ascoviridae , which suggests that the original Physcomitrella viruses were more closely related to these NCLDV families. Nevertheless, the exact phylogenetic relationships between the Physcomitrella viruses and other NCLDV families need to be confirmed when more viral sequences will be available because accelerated evolution in the NCLDV-like sequences that have most likely become non-functional after integration into the host genome can potentially cause long-branch attraction and other artefacts of phylogenetic analysis. Interestingly, the phylogenetic trees for RP1n and RP1c constructed using the same set of homologous sequences (except that we used either archaeal RP1 α′ or α′′ subunits as outgroup, respectively) were broadly consistent between each other except for deeper nodes that were not well resolved in both trees ( Fig. 4 ). Both the P. patens RP1n and RP1c proteins had similar phylogenetic affinity with the two halves of the same RP1 proteins from Iridoviridae and Poxviridae , which supports the hypothesis that RP1n and RP1c genes derived from fission of the same ancestral gene and suggests that the RP1 gene split may be a signature of the viral lineage that gave rise to the NCLDV-like regions. 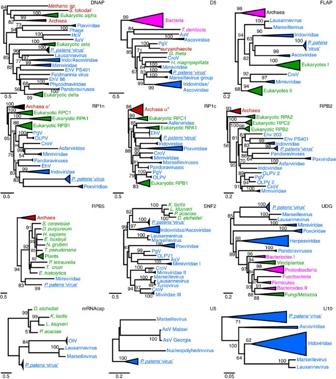Figure 4: Maximum likelihood phylogenetic trees ofP. patensNCLDV-like proteins. NCLDV, archaeal, bacterial and eukaryotic sequence names are shown in blue, red, pink and green, respectively. Subtrees containing sequences originating from the same taxonomic clade were condensed (coloured triangles). Statistical supports for branch in percent (approximate likelihood ratio test) are shown beside nodes (only branch supports >50%). Scale bar represents the number of substitutions per amino-acid site. Note that the SSB proteins were not included in this analysis because the levels of similarity between sequences were too weak for reliable phylogenetic reconstruction. AsV, African swine fever virus; CroV,Cafeteria roenbergensisvirus; EhV, Emiliania huxleyii virus; HcV,Heterocapsa circularisquamavirus; OlV,Ostreococcus luminarusvirus; OLPDV, organic lake Phycodnavirus; PgV,Phaeocystis globosavirus. Figure 4: Maximum likelihood phylogenetic trees of P. patens NCLDV-like proteins. NCLDV, archaeal, bacterial and eukaryotic sequence names are shown in blue, red, pink and green, respectively. Subtrees containing sequences originating from the same taxonomic clade were condensed (coloured triangles). Statistical supports for branch in percent (approximate likelihood ratio test) are shown beside nodes (only branch supports >50%). Scale bar represents the number of substitutions per amino-acid site. Note that the SSB proteins were not included in this analysis because the levels of similarity between sequences were too weak for reliable phylogenetic reconstruction. AsV, African swine fever virus; CroV, Cafeteria roenbergensis virus; EhV, Emiliania huxleyii virus; HcV, Heterocapsa circularisquama virus; OlV, Ostreococcus luminarus virus; OLPDV, organic lake Phycodnavirus; PgV, Phaeocystis globosa virus. Full size image Propagation of P. patens NCLDV-like regions Two mechanisms can explain the propagation of the NCLDV-like regions into the P. patens genome. They may have arisen from recurrent duplications of a single anciently integrated viral DNA by endogenous mechanisms such as unequal crossing over and heterologous recombination (Scenario S1 hereafter). Alternatively, they may result from multiple DNA insertions of distinct functional viruses (Scenario S2 hereafter). We tested which of the two alternatives best explains the pattern of accumulation of mutations in the NCLDV-like sequences. Importantly, we assumed that the viral DNA mainly evolved under no selective pressure after integration into the P. patens genome because the acquisition of a new function in the host is a rare evolutionary event; this assumption is supported by the observation that many genes in the NCLDV-like regions now exist as pseudogene (that is, ORFs contain internal stop codons, frame shifts or are truncated). We measured the strength of selective constraints that acted on genes by computing the ω = K a / K s ratio, where K a is the number of nonsynonymous substitutions per nonsynonymous site and K s is the number of synonymous substitutions per synonymous site, with ω <<1 denoting purifying selection and ω =1 indicating neutral evolution [24] . Under S1, which postulates that NCLDV-like regions resulted from duplication of already neutrally evolving DNA, ω ratios for gene are expected to be close to 1. Inversely, under S2, pre-NCLDV-like regions started to diverge as individual functional viruses and genes accumulated mutations under selective constraints during the time lapse before integration into the host genome. In this case, NCLDV-like genes are expected to have ω <1. As shown in Supplementary Table 3 , all NCLDV-like genes had ω ratio significantly <1 (likelihood ratio test; α =0.05 after Bonferroni correction), indicating that they retained footprints of purifying selection that acted after their divergence. In particular, ω <1 was obtained for both the RP1n and RP1c genes demonstrating that these sequences were indeed functional split genes rather than non-functional remnants of a disrupted ancestral RP1 gene. Overall, these results lend support to the hypothesis that NCLDV-like regions originate from multiple insertions of distinct viral DNAs. However, detailed examination of the NCLDV-like sequences indicated that propagation and divergence of the NCLDV-like regions may have involved multiple mechanisms. In some instances, the same mutation that disrupted a NCLDV-like gene was shared between different NCLDV-like regions. This suggests that the concerned sequences evolved by duplication of an original degraded NCLDV-like region (that is, scenario S1) or by gene conversion between NCLDV-like regions. Common and distinctive features of Pp NCLDV-like regions The entire moss genome sequence was cut into 1 kb DNA segments that were subsequently divided into three categories: (i) segments that are entirely contained within an annotated gene, (ii) segments that are entirely contained within a repeated sequence (that is, mainly transposable elements (TEs)), (iii) segments that are entirely contained within a NCLDV-like region. Segments with only partial or no overlap with any of the three categories were discarded. The average GC content for NCLDV-like DNA segments (34.0% GC) was similar to the average GC content for repeated sequences (34.3% GC) but lower than for genes (44.0% GC; Fig. 5a ). Thus, the NCLDV-like sequences cannot be readily differentiated from the rest of the repeated elements solely based on their GC profile. 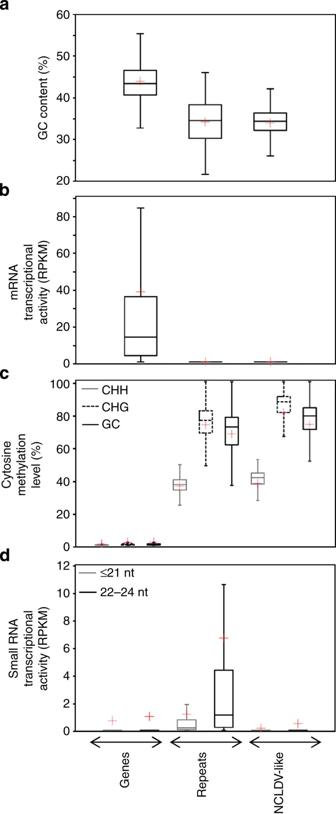Figure 5: Features ofP. patensgenomic sequences. TheP. patensgenome sequence was divided into 25,711, 133,924 and 4,261 kb segments that were entirely contained into genes, repeats and NCLDV-like regions, respectively. These genomic segments were used to measure various descriptive statistics that are summarized in box plots. Bottom and top of the box are the first and third quartiles, and the band inside the box is the median. Lines extending vertically from the boxes represent the minimum and maximum of the data. The red cross indicates the mean. (a) Box plot distributions of GC content of segments. (b) Box plot distributions of RPKM values representing average mRNA transcriptional activity of segments. RPKM values were computed from combined read mapping data of transcriptomes obtained in six different experimental conditions. (c) Box plot distributions of average cytosine methylation levels for segments. Distributions for three sequence contexts of cytosine methylation (that is, CHH, CHG and CG) are shown separately. (d) Box plot distributions of RPKM values representing small-RNA transcriptional activity in segments measured in 10-day-old protonemata. Figure 5: Features of P. patens genomic sequences. The P. patens genome sequence was divided into 25,711, 133,924 and 4,261 kb segments that were entirely contained into genes, repeats and NCLDV-like regions, respectively. These genomic segments were used to measure various descriptive statistics that are summarized in box plots. Bottom and top of the box are the first and third quartiles, and the band inside the box is the median. Lines extending vertically from the boxes represent the minimum and maximum of the data. The red cross indicates the mean. ( a ) Box plot distributions of GC content of segments. ( b ) Box plot distributions of RPKM values representing average mRNA transcriptional activity of segments. RPKM values were computed from combined read mapping data of transcriptomes obtained in six different experimental conditions. ( c ) Box plot distributions of average cytosine methylation levels for segments. Distributions for three sequence contexts of cytosine methylation (that is, CHH, CHG and CG) are shown separately. ( d ) Box plot distributions of RPKM values representing small-RNA transcriptional activity in segments measured in 10-day-old protonemata. Full size image We successfully mapped 71.4 × 10 6 mRNA-seq reads onto the moss genome, representing publicly released transcriptomes obtained in six different experimental conditions (see Methods). The read counts for the six transcriptome data sets were combined and the number of reads per kilobase per million (RPKM) mapped reads assigned to each DNA segment was used as a proxy for general expression activity. As shown in Fig. 5b , the gene DNA category exhibits a wide range of RPKM values reflecting different transcription levels. Average RPKM value for gene DNA segments was avRPKM=38.2. In contrast, repeated and NCLDV-like sequences were virtually devoid of mapped reads (avRPKM=0.14 and 0.08, respectively) indicating that these regions were globally silent under the tested experimental conditions. Some pseudogenes can go through the process of transcription, either if their own promoter is still intact or in some cases using the promoter of a nearby gene [25] . We therefore investigated possible reasons for the extensive silencing of the NCLDV-like regions. Methylation of cytosine residues is generally associated with gene transcriptional silencing in eukaryotes [26] . A previous bisulfite-seq study showed that moss TEs were highly cytosine-methylated in the CG, CHG and CHH sequence contexts (where H is A, T or C), whereas genes have little methylation in general [27] . Using the same bisulfite-seq data set, we investigated the methylation status in the three defined DNA categories. Expectedly, levels of cytosine methylation were consistent with previous results: gene segments had almost no methylated cytosines (that is, average values of 0.5% CHH, 0.6% CHG and 0.6% GC in the category), whereas repeated sequences showed much higher average frequencies of cytosine methylation in all contexts (that is, 36.3% CHH, 72.8% CHG and 66.8% GC; Fig. 5c ). Cytosine methylation patterns for NCLDV-like regions closely resemble those of repeated sequences in all contexts, suggesting that cytosine methylation might be involved in the transcriptional silencing of NCLDV-like genes. In plant genomes, DNA methylation may be directed by short interfering (si) RNA molecules that guide the de novo methylation machinery to complementary genomic DNA. siRNAs are estimated to direct approximately 30% of the cytosine methylation in Arabidopsis thaliana [28] . Signals for the remaining methylation remain to be fully defined. In moss, genomic hotspots of 22–24 nt siRNAs production were found to be depleted in gene content and enriched in TEs, suggesting that this class of siRNA has a major role in directing de novo cytosine methylation to this class of repeated sequences [29] . To test the hypothesis that the same mechanism is responsible for cytosine methylation in NCLDV-like regions, we mapped a previously reported small RNA-seq data set [29] onto the moss genome. This data set contained various families of small RNAs (19–26 nt) isolated from wild-type P. patens protonema culture, including siRNAs and microRNAs. Consistent with previous reports, repeated sequences had, on average, a relatively high number of small RNA-seq reads, the majority of which were in the 22–24 nt size class (that is, avRPKM ≤21 nt =1.16 and avRPKM 22–24 nt =6.66; Fig. 5d ). On average, gene sequences and NCLDV-like regions matched with a much smaller number of small RNAs (avRPKM ≤21 nt =0.66 and avRPKM 22-24 nt =0.98 for gene sequences and avRPKM ≤21 nt =0.13 and avRPKM 22−24 nt =0.45 for NCLDV-like regions). This result suggests that in contrast to repetitive elements, cytosine methylation in NCLDV-like regions is directed by a mechanism that does not involve the RNA-dependent DNA methylation machinery. The existence of genes from different domains of life in the NCLDV genomes has given these viruses a reputation as ‘gene robbers’ [30] , [31] . It is apparent that a number of genes have entered NCLDV genomes via horizontal transfer from their hosts, bacterial endosymbionts and also possibly from other viruses [8] , [32] . However, the extent of gene acquisitions by viruses is highly debated and may have been overestimated [33] . Here we analysed viruses and their hosts under a reverse angle. Some viruses can have their genome integrated into the genome of their host, either by an active process (for example, lysogenic cycle) or accidentally [34] , [35] . We postulated that the footprints left by these insertions, in the form of sequences with apparent viral origin, provide circumstantial evidence of past physical contact between virus and plants, presumably through infection. We have implemented a method that permits identification of genes that have a potential viral origin in a plant genome. Remarkably, only the two early diverging land plant species, namely P. patens and S. moellendorffii , were found to contain NCLDV-like genes. Although a lack of evidence cannot be taken as a proof of absence, it is possible that the seed plants, to which belong the 11 remaining species, developed strategies that hamper NCLDV endogenization or protect them from infection. For instance, the prolonged haploid stage in the life cycle of bryophytes and lycophytes may constitute a period of vulnerability to viral insertions; whereas the microspore haploid stage is relatively short in seed plants reproduction cycle. Additional plant genomes are currently being sequenced including members of the spore-reproducing ferns and embryophytes, which will allow further assessment of the taxonomic distribution of endogenous NCLDVs in plants. However, an important finding of our analysis is that at least some land plants were likely infected by unknown NCLDV members. Only a single S. moellendorffii gene family, encoding exoribonuclease, had a clear origin in NCLDV. The mechanism by which this gene family was incorporated and propagated in the Selaginella genome is unknown. Molecular evolution analysis indicated that the Selaginella sequences evolved under purifying selection after their divergence ( ω <<1; see Supplementary Table 3 ). However, it is unclear whether the footprints of selection reflect functional constraints that occurred in donor viruses before multiple gene insertions (that is, scenario S2) or in S. moellendorffii after an inserted viral gene gained a new biological function beneficial to the host and was duplicated afterwards. Although P. patens NCLDV-like genes also have ω <<1, this latter scenario was not considered for P. patens NCLDV-like regions because the gain of a new function is a rare evolutionary event and it is therefore unlikely that 16 clustered viral genes gained a new function at the same time. The discovery of NCLDV-like regions in the P. patens genome also raises many questions. First, it is unclear whether the 20 NCLDV-like gene families represent the complete gene repertoire of original P. patens viruses. Sequenced NCLDVs have much larger genomes than the estimated 13 kb of the reconstructed original region. For instance, the smallest known NCLDV genome is that of Lymphocystis disease virus 1 ( Iridoviridae ), which is 103 kb and encodes 110 predicted proteins [36] . On the other side of the size scale, Pandoraviruses have genomes up to 2.5 Mb and 2,556 putative protein-coding sequences [13] . The fact that NCLDV-like regions contain a dense, redundant assemblage of NCLDV core genes that are interrupted by only few orphan genes suggests that the genome and gene set of original viruses may be extraordinarily small among NCLDVs. However, the P. patens NCLDV-like regions lacked core genes that encode essential components of DNA replication in NCLDVs, such as DNA ligases, topoisomerases and DNA sliding clamps. Other absences are genes encoding particle structural components, such as the major capsid protein and packaging ATPase, which are hallmarks of large eukaryotic dsDNA viruses that have icosahedral symmetry (for example, excludes Poxviruses and Pandoraviruses). Thus, although we cannot exclude that fast-evolving viral genes were missed outside of NCLDV-like regions during our analysis, the reconstructed NCLDV-like gene complement is unlikely to enable a virus to complete a full replication cycle, including particle assembly. This suggests that the original P. patens viruses relied on a larger set of proteins from its host and/or co-infecting virus. Alternatively, NCLDV-like regions could originate from recurrent insertion of the same homologous DNA fragments from larger, autonomous virus genomes. Another possibility accounting for the absence of certain core NCLDV genes is that the most recent common ancestor of the NCLDV-like regions was not a virus. Some fungi and plants harbour linear DNA plasmids in their mitochondria [37] . These replicons range from 2 to 13 kb in size and contain 2–6 ORFs, including ORFs encoding DNA and/or RNAPs that are phylogenetically related to bacteriophages and adenoviruses. The NCLDV-like regions, which also encode DNAPs and various RNAP subunits, may be remnants of analogous mitochondrial linear plasmids integrated into the Physcomitrella nuclear genome. However, this hypothesis is unlikely for two reasons. First, NCLDV-like regions contain a set of ORFs that are involved in DNA replication and repair, mRNA maturation and transcription, which are characteristic of NCLDVs but absent in known linear plasmids. Second, DNA and RNAPs encoded in mitochondrial linear plasmids only present very weak sequence similarity, almost below detectable levels, with NCLDV-like proteins and NCLDV homologues in general. This indicates that plant linear plasmids and NCLDV-like regions are remotely phylogenetically related. We also considered the hypothesis that the NCLDV-like regions are inactivated copies of a novel TE related to NCLDV. The nature of genes contained in the NCLDV-like fragments tends to argue against this possibility. There are seven genes involved in transcription and mRNA maturation. These genes are almost exclusively found in NCLDVs that replicate in the host cytoplasm. NCLDVs that replicate in the host nucleus (for example, Chloroviruses, Prasinovirus) have lost these genes (except mRNA capping methyltransferase and TFIIS) and rely entirely on the host RNA transcription machinery [9] . Thus, it appears unlikely that a TE, a resident of the nucleus, encodes so many enzymes that are naturally present in abundance in the nucleus. Another class of enzymes that cast doubt on the TE hypothesis is the DNA repair machinery. UDG and FLAP endonucleases have systemic action and make a priori no distinction between the host genome and TEs. Thus, enzymes produced by a TE would be more occupied to repair the host genome (that is quantitatively over dominant) than the TE itself. It appears unlikely that evolution selects such inefficient genetic combination. Last, we found no evidence that the NCLDV-like fragments encode an integrase and we found no terminal repeats or duplicated integration sites. Although our data suggests that the moss NCLDV-like regions have a NCLDV origin, the nature of viruses that gave rise to them remains to be elucidated. Nevertheless, even though the infectious cycle of donor viruses is unknown, a complex complement of transcription-related genes suggests that the ancestral P. patens virus most likely replicated in the host cytoplasm, which is a common feature of NCLDVs. Overall, our work illustrates how the study of plant endogenous viruses can bring significant insights into the understanding of the plant virome and viral host range. It highlights the need for comprehensive analyses of viral footprints in eukaryotic genomes, which are likely to help to better understand host–virus interactions and the evolutionary impacts of viral inserts in host genomes. For instance, endogenized viral genes can be domesticated towards cellular functions [38] , and viral material can have a role in immunity against environmental viruses [39] , [40] . In addition, viruses are acknowledged as vectors of HGT and a recent study provided convincing evidence that baculoviruses mediate the horizontal transfer of TEs between eukaryotes [41] . Thus, a variety of interactions that regulate plant populations and evolution may be at play. Sequence analysis The 13 selected species are model representatives of important land plant taxonomic clades including dicot ( A. thaliana (family: Brassicaceae), Glycine max (Fabaceae) , Medicago truncatula (Fabaceae) , Populus trichocarpa (Salicaceae) , Ricinus communis (Euphorbiaceae) , Vitis vinifera (Vitaceae) , Solanum lycopersicum (Solanaceae)), monocot ( Oryza sativa (Poaceae) , Sorghum bicolor (Poaceae)), early diverging angiosperm ( Amborella trichopoda (Amborellaceae)), gymnosperm (Picea abies (Pinaceae)), bryophyte ( P. patens (Funariaceae)) and lycophyte ( S. moellendorffii (Selaginellaceae)). Genome sequences and annotations were downloaded from http://www.amborella.org/ ( A. trichopoda assembly V1.0), http://congenie.org/ ( P. abies assembly V1.0) and the phytozome v9.1 database [42] (containing the following annotation versions: A. thaliana TAIR release 10 , G. max Glyma1.1 , M. truncatula Mt3.5v4 , P. trichocarpa JGI annotation v3.0, R. communis TIGR release 0.1 , V. vinifera March 2010 12X assembly and annotation from Genoscope , S. lycopersicum ITAG2.3, O. sativa MSU release 7.0 , S. bicolor Sbi1.4 models from MIPS/PASA, P. patens COSMOSS annotation v1.6 and S . moellendorffii JGI annotation v1.0 ). Plant proteins were aligned against the Genbank NR database using BLASTP. Only hits with E -value <1e−5 were considered significant. For each protein, the sequences of the best hit among NCLDVs and the best hit among cellular organisms that do not belong to the same family (that is, the taxonomic rank) as the query were downloaded. The hit and query sequences were realigned against the query in another BLASTP round, but this time by deactivating the option of masking low complexity regions (-F F). The resulting scores were used to calculate the relative-scores in Fig. 1 . To confirm that the absence of NCLDV-like gene candidates in Embryophytes was not due to missannotation of viral sequences, we masked the regions of genomes that corresponded to predicted coding sequences. Then, ORFs >90 codons were extracted from the non-masked regions (which potentially includes unannotated ORFs and degraded ORFs) and treated the same way as for predicted proteins to construct similarity plots. A number of plant ORFs significantly matched with NCLDV-encoded proteins, the majority of which were related to TE proteins. However, similarity plots indicated that these ORFs were more similar to plant homologues than to NCLDV homologues ( Supplementary Fig. 18 ). Thus, we can be confident that the studied Embryophyte genomes are free from NCLDV-like gene candidates. Identification and analysis of the P. patens NDLDV-like regions were conducted using version 1.6 of the moss genome assembly [43] . The DNA sequences around the candidate NCLDV-like genes were extracted and regions of high sequence similarity between each other were identified using dot plot alignments. The two longest similar regions containing NCLDV-like genes were precisely delimited, manually annotated, masked for TEs and served as reference in an initial BLASTN search against the P. patens genome (-F F). Additional NCLDV-like regions were identified by considering hits with a high level of similarity (that is, >80% identity) and E -value <1e−40. The sequences of the newly identified NCLDV-like regions were extracted, masked for TEs and added to the query set. Rounds of BLASTN alignments against the genome (-F F), identification of new NCLDV-like regions, sequence extraction, repeat masking and inclusion into the query set were repeated until no new NCLDV-like regions were identified or extended. The coordinates of the final BLASTN alignments were used to precisely delimit the borders of NCLDV-like regions. Reannotation of NCLDV-like regions in Physcomitrella and Selaginella was performed using a combination of standard ORFing procedure (ORFs >90 codons) and GENEWISE predictions using NCLDV proteins as guide [20] . Repeated sequences analysed in Fig. 5 were defined as non-gene sequences with five or more BLASTN matches in the P. patens genome ( E -value <1e−40 and –F F). We used BLAST against the NCBI database to collect the presence/absence taxonomic distribution reported in Supplementary Table 1 . We used Position-Specific Iterated BLAST to search for homologues of the putative SSB proteins from moss NCLDV loci in the NCBI database. RNA-seq and BS-seq data were downloaded from the Gene Expression Omnibus (GEO) database. GEO accession numbers are GSE36274 (mRNA-seq; red light response [44] ), GSE25237 (mRNA-seq; DNA damage response), GSE18466 (small RNA-seq; 10-day-old protonemata [28] ) and GSM497264 (bisulfite sequencing; DNA methylation in P. patens [26] ). Small-RNA-seq reads were aligned onto the moss genome assembly V1.6 with the BLASTN programme. Only matches over the entire length of reads and no mismatch in the alignment were considered. mRNA-seq reads were mapped with the BOWTIE2 programme [45] allowing at most two mismatches with the genome sequence. When pair-end reads were available, we only mapped one read of each pair. For the DNA methylation data analysis, we directly used the results of BS-seq read mapping obtained by the authors of the initial study [26] that were available as part of the GEO entry. Phylogeny Construction of adequate homologous protein sets for phylogenetic analysis was performed using the BLAST-EXPLORER website [46] . Homologous proteins were aligned using MUSCLE [47] and amino-acid positions in multiple-alignments containing gaps were removed. ML phylogenetic reconstruction was performed using the PHYML programme [48] . Before phylogenetic reconstruction, the best fitting substitution model for each sequence data set was determined using the PROTTEST programme [49] . Alignments are available in Supplementary Data 1–14 . Molecular evolution Because the LTRs from LTR retrotransposons (LTR-RTs) are identical upon insertion and then accumulate mutations neutrally over time, their divergence is indicative of integration time [50] . LTR-RTs were searched in moss NCLDV-like loci using LTRharvest [51] . Each LTRharvest prediction was compared with the Repbase database for validation and classification. All eight true positives were Gypsy-like elements. From these, each pair of LTRs was retrieved and aligned using MUSCLE [47] , and evolutionary distances were calculated with ‘Distmat’ from the Emboss package [52] using the Kimura two-parameter model. Distances per site were then transformed into ages by applying an average rate of 1.3 × 10 −8 substitution per site per year as estimated previously from plant neutrally evolving DNA [53] ( Supplementary Table 2 ). This same calibration was used to infer the age of LTR-RT activity in P. patens [54] . Analysis of the ratio ω = K a / K s was done using a ML approach implemented in the CODEML programme [55] . We analysed aligned codon sequences using two variants of the one-ratio model (M0). In a first CODEML run, the M0 model was set so that ω is freely estimated from the data. To test the null hypothesis that the estimated ω is equal to 1, we ran CODEML a second time with ω fixed to 1 and applied the likelihood ratio test: twice the log-likelihood difference between the two variant models (2ΔlnL=2 × [lnL ω =free −lnL ω =1 ]) was compared with a χ 2 distribution with one degree of freedom. Plant material and culture conditions The Gransden, Honnef and Uppsala-K1 wild-type strains of P. patens ( http://www.moss-stock-center.org/ ), wt4 wild-type strain of Ceratodon purpureus [56] and wild-type strain of Pseudocrossidium replicatum (gift of Dr Villalobos, CIBA-IPN, Tlaxcala, Mexico) were used in this study. Protonemal tissues were vegetatively propagated as previously described [57] . Molecular analysis Genomic DNA was isolated from protonemal tissue as previously described [57] . Using genomic DNA as starting template, we amplified PCR fragments covering the NCLDV domains D5, TFIIS, RPB2 and the genomic locus adenine phosphoribosyl transferase. PCR amplifications were performed using 0.5 ng moss genomic DNA in a 50-μl reaction mix containing 5 μl PCR DreamTaq Buffer (Thermo Scientific), 1.25 U DreamTaq DNAP (Thermo Scientific), 0.2 mM dNTPs and 0.8 μM of each primer. The thermal cycling conditions were as follows: 1 min denaturation at 94 °C; 30 cycles of 30 s denaturation at 94 °C, 30 s annealing at 58 °C and 1 min extension at 72 °C; and a final 3 min extension at 72 °C. The primers used in this study are described in Supplementary Table 4 . F.M. and G.B. designed and coordinated the project, performed bioinformatic analyses and wrote the paper. A.E. and F.N. performed PCR analyses and wrote the corresponding section. How to cite this article: Maumus, F. et al . Plant genomes enclose footprints of past infections by giant virus relatives. Nat. Commun. 5:4268 doi: 10.1038/ncomms5268 (2014).